Unravelling the biodiversity of nanoscale signatures of spider silk fibres Living organisms are masters at designing outstanding self-assembled nanostructures through a hierarchical organization of modular proteins. Protein-based biopolymers improved and selected by the driving forces of molecular evolution are among the most impressive archetypes of nanomaterials. One of these biomacromolecules is the myriad of compound fibroins of spider silks, which combine surprisingly high tensile strength with great elasticity. However, no consensus on the nano-organization of spider silk fibres has been reached. Here we explore the biodiversity of spider silk fibres, focusing on nanoscale characterization with high-resolution atomic force microscopy. Our results reveal an evolution of the nanoroughness, nanostiffness, nanoviscoelastic, nanotribological and nanoelectric organization of microfibres, even when they share similar sizes and shapes. These features are related to unique aspects of their molecular structures. The results show that combined nanoscale analyses of spider silks may enable the screening of appropriate motifs for bioengineering synthetic fibres from recombinant proteins. Spiders are one of the most impressive tailors of the biological world and have long fascinated laypersons and scientists. The number of scientific papers and patents that describe the structure and/or function of spider silk has increased exponentially over the last 20 years, as has the number of citations of these publications (see Supplementary Fig. 1 ). This great interest stems from the fact that spiders produce up to seven different high-performance protein-based types of silk fibres with a variety of mechanostructural and functional attributes [1] . The primary structures of spider silk proteins (spidroins) consist mostly of the amino acids alanine, glycine and serine, which are organized into motifs that exhibit a high secondary structure content characterized by antiparallel β-sheets (crystal domains) and β-turns (amorphous domains) that exhibit outstanding mechanical properties [1] , [2] . Crystal domains are commonly associated with repeating poly(alanine) units or repeating motifs in which glycine alternates with either alanine or serine; amorphous domains are glycine-rich domains [2] , [3] . To date, computational calculations [4] , X-ray diffraction [5] , nuclear magnetic resonance [6] , polarized light microscopy [7] , scanning electron microscopy [7] , [8] , transmission electron microscopy [9] , Raman spectromicroscopy [10] and, more recently, atomic force microscopy (AFM) [11] , [12] , [13] , [14] , [15] , [16] , [17] have been the most commonly used techniques to study the nanoarrangements of silk fibre domains. However, the details of the size, topology, mechanical features and fractional composition of the crystalline and amorphous domains remain to be clarified. In addition, although more than 40,000 spider species have been identified, fewer than one dozen have been investigated in terms of the hierarchical composition of silk fibres and the organization of protein modules. With the advent of AFM, researchers are now pursuing investigations of the structural and mechanical nanodomains of spider silks, particularly in their near native condition. Previous investigations of the nanostructure of spider silks by AFM focused on the qualitative topographical imaging of sectioned [11] , dissociated [12] , reassembled [13] or synthetic [14] silk fibres. In this study we explore the surface of natural spider silk fibres simply rolled around a solid graphite substrate, which could more roughly reflect the bulk properties of these biomaterials. Towards this end, with the advent of several secondary AFM imaging modes that offer unprecedented nanoscale spatial resolution and high sensitivity for the detection of properties due to compositional/chemical variations of elastomeric materials, we also mapped local frictional, stiffness, viscoelastic and surface potential properties of spider silks ( Fig. 1a ). This strategy is congruent with an array of evidence that indicates that surface topography is directly related to other intrinsic material properties [18] . 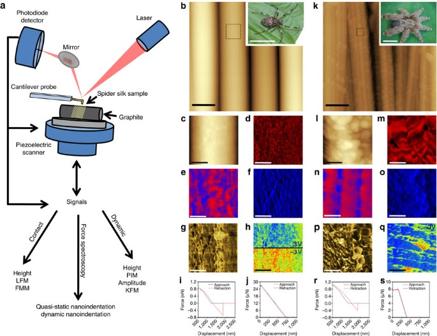Figure 1: Overview of AFM techniques used to characterize spider silk fibres. (a) Schematic representation of the experimental drawing. (b,c,k,l) Height images showing surface variations over the areas. The insets in panelsbandkare photos ofN. cruentata(Ncru) andA. juruensis(Ajur) specimens, respectively. (d,m) Lateral force images showing the frictional forces between the silk fibre components and the AFM probe, contrasting low (black) and high (red) friction. (e,n) Force modulation images showing the stiffness of the silk fibres, contrasting soft (blue) and stiff (red) areas. (f,o) Amplitude images showing the edges of the silk fibre components. (g,p) Phase images showing the viscoelasticity of the silk fibres resolved with high spatial resolution as well as the compositional/mechanical variations between crystalline (brown to black) and amorphous (golden to yellow) domains. (h,q) Kelvin probe force images showing the surface potential of the silk fibres according to the voltage bias applied. (i,r) Conventional force curves. (j,s) Dynamic force curves. Left panels (Ncru) and right panels (Ajur). Barsbandk=1 μm,c–h=200 nm andl–q=100 nm. Inset bars=20 mm. The represented areas do not match exactly due to the expected misregistration among multiple AFM acquisition modes, except forcandldetailed view that match exactly the area surrounded by black squares onbandkimages. Force modulation microscopy (FMM); Phase imaging microscopy (PIM). Figure 1: Overview of AFM techniques used to characterize spider silk fibres. ( a ) Schematic representation of the experimental drawing. ( b , c , k , l ) Height images showing surface variations over the areas. The insets in panels b and k are photos of N. cruentata ( Ncru ) and A. juruensis ( Ajur ) specimens, respectively. ( d , m ) Lateral force images showing the frictional forces between the silk fibre components and the AFM probe, contrasting low (black) and high (red) friction. ( e , n ) Force modulation images showing the stiffness of the silk fibres, contrasting soft (blue) and stiff (red) areas. ( f , o ) Amplitude images showing the edges of the silk fibre components. ( g , p ) Phase images showing the viscoelasticity of the silk fibres resolved with high spatial resolution as well as the compositional/mechanical variations between crystalline (brown to black) and amorphous (golden to yellow) domains. ( h , q ) Kelvin probe force images showing the surface potential of the silk fibres according to the voltage bias applied. ( i , r ) Conventional force curves. ( j , s ) Dynamic force curves. Left panels ( Ncru ) and right panels ( Ajur ). Bars b and k =1 μm, c – h =200 nm and l – q =100 nm. Inset bars=20 mm. The represented areas do not match exactly due to the expected misregistration among multiple AFM acquisition modes, except for c and l detailed view that match exactly the area surrounded by black squares on b and k images. Force modulation microscopy (FMM); Phase imaging microscopy (PIM). Full size image Nanoscale imaging of spider silk fibres Representative AFM images obtained in sample areas in which parallel silk fibres of two phylogenetically distant spiders are shown in Figs 1 and 2 (see Supplementary Fig. 2 for all species investigated). The height images at wide field ( Figs 1b,k and 2a,b , and Supplementary Fig. 2 ) displayed clearly distinct silk fibre diameters according to spider species (see Supplementary Fig. 3a ), in good agreement with previous scanning electron microscopy and polarized light microscopy data [7] . The height images at higher magnification also revealed meaningful differences in the two-dimensional roughness of the spider silk fibres, at least when phylogenetically distant species were compared ( Figs 1c,l and 2c,d , and Supplementary Fig. 3b ). However, some features, such as the numerous nanofibrils formed by heterogeneous protrusions arranged in the direction of the fibres, are slightly more resolved and contrasted in the lateral force microscopy (LFM) and amplitude images ( Fig. 1d,f,m,o ) because these two acquisition modes map the friction and slope/edges of the sample, respectively. The force modulation microscopy technique revealed differences in the local deformation/stiffness properties of the silk fibres ( Fig. 1e,n ), suggesting the presence of harder (red areas, most likely crystal domains) and softer (blue areas, most likely amorphous domains) structures, although it is not possible to rule out some type of surface topographic influence. 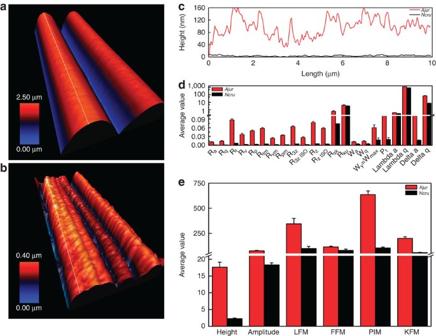Figure 2: Overview of AFM topographical three-dimensional patterns obtained from fibres of two spider species. (a)N. cruentata(Ncru) and (b)A. juruensis(Ajur). Both 3D perspective images are shown with displayed areas of 5 × 10 μm. (c)NcruandAjurheight profiles following the white dashed line drawn inaandb. (d)NcruandAjuramplitude (Ra, Rq, Rt, Rv, Rm, Rp, Rtm, Rvm, Rpm, R3z, R3zISO, Rz, RzISO, Rsk, Rku, Wa, Wq, Wyand Pt), spatial (lambda a and lambda q), and hybrid (delta a and delta q) one-dimensional standard roughness profile parameters. (e)NcruandAjurnanoroughness (height), nanoedge (amplitude), nanotribological (LFM), nanostiffness (FFM), nanoviscoelasticity (PIM) and nanoelectrical (KFM) parameters expressed as average values. All parameters revealed statistically significant differences between the two species at aP<0.01. Figure 2: Overview of AFM topographical three-dimensional patterns obtained from fibres of two spider species. ( a ) N. cruentata ( Ncru ) and ( b ) A. juruensis ( Ajur ). Both 3D perspective images are shown with displayed areas of 5 × 10 μm. ( c ) Ncru and Ajur height profiles following the white dashed line drawn in a and b . ( d ) Ncru and Ajur amplitude (R a , R q , R t , R v , R m , R p , R tm , R vm , R pm , R 3z , R 3zISO , R z , R zISO , R sk , R ku , W a , W q , W y and P t ), spatial (lambda a and lambda q), and hybrid (delta a and delta q) one-dimensional standard roughness profile parameters. ( e ) Ncru and Ajur nanoroughness (height), nanoedge (amplitude), nanotribological (LFM), nanostiffness (FFM), nanoviscoelasticity (PIM) and nanoelectrical (KFM) parameters expressed as average values. All parameters revealed statistically significant differences between the two species at a P <0.01. Full size image To observe the inner layers of the spider silk fibres, the hard tapping mode (dynamic) was used to penetrate the surface and reveal viscoelastic details of the hierarchical organization of the silk domains while avoiding any influence from the outer layers of the fibre surface [11] . In contrast to other AFM modes, tiny features of the fibres were clearly resolvable in viscoelastic (phase imaging microscopy) images ( Fig. 1g,p ). Because spider silks contain two main molecular phases (amorphous and crystalline), each with a possible range of organizational states (from unordered to well-ordered) [1] , phase images provided a map of stiffness and viscoelastic variations in the sample that could be associated with these molecular phases. Although the conservation of nanostructured protein motifs confers extraordinary mechanical attributes to spider fibres leading to robust webs [19] , spider fibres are also recognized as poor conductors of electricity [20] . However, spider silk fibres have been suggested to be susceptible to electrostatic cling [21] , similar to that observed for several synthetic polymeric materials, although this suggestion has not been supported experimentally on the macroscale [22] . Thus, Kelvin force microscopy (KFM) was used to directly image differences in the surface nanopotential of the fibres. When the voltage bias was swept from positive (3 V) to negative (−3 V), a particular image with variable potential surface contrast appeared on silk fibres depending on the relative sign of the charge ( Fig. 1h ). However, because both sample bias polarities resulted in similar general profiles, a negative potential was chosen for comparison purposes among fibres ( Fig. 1q ). The detected signal may have been due to the very low content of charged acidic and basic amino acid residues or other biomolecules, such as lipids, on the surface of the silk fibres. Comprehensive quantitative mapping of spider silk fibres In addition to the surface topography, the present study has utilized a variety of AFM acquisition modes to nanoimage spider silk fibres that combine topographical, tribological, mechanical (stiffness and viscoelasticity) and surface electrostatic potential mapping at the highest possible resolution. Therefore, our acquired data sets for each spider species contain a large number of images that provide a huge quantity of information about the fibres that should be quantitatively rationalized. Although nanoscale features from images acquired by AFM can be quantitatively measured in several different ways, we chose to measure the longitudinal line profile nanoroughness ( Fig. 2d ), the surface nanoroughness (see Supplementary Fig. 3b ) and the average value of the nanoscale features ( Fig. 2e and Supplementary Fig. 4 ) of the spider silk fibres that exhibited distinguishable features mainly in unrelated species. However, other researchers may experience difficulty in reproducing our experiments with exactly the same instrumental setup (for example, environmental conditions or probe mechanics) due to interspecific, intraspecific and intraindividual variations as well as the presence of fibre nanodomains, for example, the presence of gum-like substances (see Supplementary Fig. 5 ). Therefore, we avoided reporting absolute quantities and instead relied on normalized values and ratios during comparisons among fibres. Because a comparison of thousands of images by eye or the construction of plots for all fibre absolute values is unfeasible, we used the root mean square (RMS) mean value as the quantitative statistical parameter to characterize and compare acquisition-mode data among fibres. Thus, the high RMS average values are likely abrupt fluctuations due to extremes in the descriptors at the nanoscale. However, the low RMS average values strongly indicate regular surfaces at the nanoscale. We also used the relative standard error of the mean RMS (RSERMS) as the measure of variation within our data set and, consequently, among regions of these fibres. 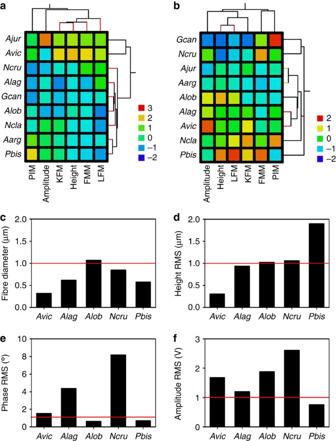Figure 3: Permuted data matrix maps of hierarchical cluster analyses. (a) RMS and (b) RSERMS of spider silk fibres and AFM acquisition modes. Red-orange, green and blue cells represent a high, moderate and low relative content/value of each analysed parameter, respectively. Each cell in the colour matrices represents the average value for 15 scanned areas of one fibre for a given AFM mode. Colour gradients represent the normalization of the compared data. Dendrograms at the right side of the matrices represent the relationship between the spider silk fibres, and the upper dendrograms indicate relationship between AFM acquisition modes. The distance function is based on Euclidean distance. (c) Diameter; (d) height root mean square (RMS); (e) phase RMS and (f) amplitude RMS of fresh (0 day) and aged (1-year-old) silk fibres from five spider species. Red lines indicate the normalized value based on 0 day (value 1). Figure 3a and b illustrate the overall RMS and RSERMS data, respectively, which were obtained from normalized permuted data colour matrix maps of Hierarchical cluster analyses (HCA) of spider silk fibres investigated under different AFM modes. Figure 3: Permuted data matrix maps of hierarchical cluster analyses. ( a ) RMS and ( b ) RSERMS of spider silk fibres and AFM acquisition modes. Red-orange, green and blue cells represent a high, moderate and low relative content/value of each analysed parameter, respectively. Each cell in the colour matrices represents the average value for 15 scanned areas of one fibre for a given AFM mode. Colour gradients represent the normalization of the compared data. Dendrograms at the right side of the matrices represent the relationship between the spider silk fibres, and the upper dendrograms indicate relationship between AFM acquisition modes. The distance function is based on Euclidean distance. ( c ) Diameter; ( d ) height root mean square (RMS); ( e ) phase RMS and ( f ) amplitude RMS of fresh (0 day) and aged (1-year-old) silk fibres from five spider species. Red lines indicate the normalized value based on 0 day (value 1). Full size image Silk fibres-based nanoscale phylogeny of spiders From the RMS data ( Fig. 3a ), the upper dendrogram of the matrix in Fig. 3a represents an innovative means of comparing AFM acquisition modes to characterize materials. AFM modes such as KFM, LFM and force modulation microscopy exhibit a noticeably strong correlation with the height mode and appear to be influenced by the topography of the sample, as has been qualitatively argued by others [23] . In addition, the dendrogram at the right side of the matrix shows that silk fibres from spiders with a common evolutionary origin are distinctly clustered together into the infraorders Mygalomorphae ( Ajur and Avic ) and Araneomorphae (other species investigated). This result was not surprising given that Mygalomorphae diverged from Araneomorphae spiders and, consequently, from their silk fibre spidroins, at least 240 Myr ago [24] . However, the novelty is that the nanoscale features of silk fibres per se provided us with signatures similar to those obtained by well-established available taxonomic classification methods, that is, those based on anatomical character and DNA sequence comparisons. This approach opens a plethora of new research directions in the field of high-throughput bioprospecting of fibres with desirable physical properties, without prior knowledge of their DNA or protein sequences. Although estimators of data variation (for example, RSERMS) are commonly used in association with central tendency measurements (for example, RMS average values), they can also be individually plotted to reveal noticeable variations among sampled areas. From the RSERMS data ( Fig. 3b ), the broad range of values observed for different spider species and AFM modes indicates that, although some fibres may be homogeneous for a certain nanoscale features, they could be strongly heterogeneous for other properties as well. Therefore, the dendrogram at top of the matrix in Fig. 3b provides a measure of the relatedness of the AFM modes according to their RSERMS, which showed that the height and LFM modes exhibit similar variations. In addition, the dendrogram at the right side of the matrix in Fig. 3b shows that the spider silk fibres clustered into groups with no apparent evolutionary or functional attribute. These results are in agreement with those of other studies and show that variations in the spider silk fibre properties (for example, strength or toughness) fall within a wide order of magnitude within and across species [7] , [25] , [26] . This intriguing phenotypic plasticity of silks has been associated with a spider’s weight [27] , spinning conditions [28] , prey type [29] , environment [30] , parasitoids [31] and age [32] rather than any phylogenetic attribute. Ageing effects on nanoscale features of spider silk fibres AFM imaging of the same spider silk fibres 1 year after the first measurements revealed that only some significant mechanostructural differences ( P <0.05) occurred in the diameter, height RMS, phase RMS and amplitude RMS ( Fig. 3c and Supplementary Fig. 6 ). Increases or decreases in parameter values as a result of ageing may reflect the hydration state [32] , [33] , the salt/shear [34] , the molecular rearrangement [35] or the degradation of some outer/inner layer [36] of the silk fibres. It is reasonable to speculate that more than one of these phenomena may be important. Nevertheless, the lack of any reliable pattern among spider species with respect to the observed differences between fresh and aged fibres is notable. This fact contrasts with published data indicating that 1 year of benign aging consistently resulted in a decrease in the diameter of spider silk fibres, with a trend towards an improvement in their mechanical performance [32] . We argue that this disagreement is likely due to differences among species (for example, spidroin sequences), measurement techniques or, more likely, the environmental conditions at the moment of the experiments. Other researchers [33] and we (unpublished data) have found that spider silk fibres can capture small amounts of water from humid air, which may influence any measurements. This possibility will be investigated further through a comparison of spider silk fibres aged for several years under well-controlled conditions. Nanomechanical behaviour of spider silk fibres Although traditional (height) and non-traditional (that is, LFM, FFM, phase imaging microscopy, and KFM) AFM imaging modes offer the opportunity to map the surface of silk fibres in at least three dimensions simultaneously, force spectroscopy experiments can measure intermolecular forces between an AFM probe and the fibre surface as a function of distance at unprecedentedly high resolutions. The transversal nanomechanical properties of single fibres were measured by quasi-static and dynamic AFM nanoindentation approaches ( Fig. 1i,r,j,s , respectively). In addition, there is a consensus that spider silk fibres share extraordinary mechanical properties with some of the most impressive man-made materials, and that, despite remarkable recent advances, [37] , [38] researchers are currently not able to completely biomimic such attributes in artificial fibres. Considering these points, we measured steel and nylon wires as well as synthetic fibres extruded from recombinant spidroins in a comparative manner (see Supplementary Fig. 7a–c ). We used neighbour-joining dendrograms using Euclidean distance ( Fig. 4a–c ) and principal component analysis ( Fig. 4d ) for clarity and to enable better/faster overall comparisons of the nanomechanical parameters derived from force spectroscopy data for the materials. Clear differences were observed between clustering of the spider silks due to the nanoindentation technique used and the experimental conditions. Quasi-static and dynamic nanoindentation approaches provided measurements under closed- and opened-loop load control, respectively. Both strategies indicated that spider silks from Mygalomorphae species clustered together at a low Euclidean distance. In addition, some of the other spider silks shared similarities among themselves or with man-made materials, rendering specific clades ( Fig. 4a–c ). 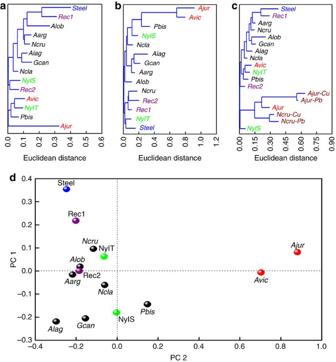Figure 4: Force spectroscopy data illustrated by multivariate statistics approaches. (a) Cladogram showing the phylogenetic relationships of spiders inferred using static nanomechanics data. (b) Cladogram showing the phylogenetic relationships of spiders inferred using dynamic nanomechanics data. (c) Cladogram showing the phylogenetic relationships of spiders inferred using static and dynamic nanomechanics data, including metal-infiltrated fibres. (d) Principal component analysis showing the phylogenetic relationships of spiders inferred using static and dynamic nanomechanics data. Figure 4: Force spectroscopy data illustrated by multivariate statistics approaches. ( a ) Cladogram showing the phylogenetic relationships of spiders inferred using static nanomechanics data. ( b ) Cladogram showing the phylogenetic relationships of spiders inferred using dynamic nanomechanics data. ( c ) Cladogram showing the phylogenetic relationships of spiders inferred using static and dynamic nanomechanics data, including metal-infiltrated fibres. ( d ) Principal component analysis showing the phylogenetic relationships of spiders inferred using static and dynamic nanomechanics data. Full size image Metal effects on nanomechanics of spider silk fibres Synthetic spider silk fibres reinforced by small amounts of metal vapours have recently been reported to show improved strength performance [39] . To determine the effects of metals on natural silk fibres, some fibres investigated in the present study were exposed to copper and lead ions, resulting in a significantly higher Young’s modulus, which corroborates the previous insight that metal ions could reinforce spider silk fibres ( Fig. 4c and Supplementary Fig. 7d ). Because this effect can also be observed in natural fibres, this could also be considered a natural phenomenon for silks tailored on metal-rich environments. Nanostructural variability of spider silk fibres Aqueous samples of silk spidroin under controlled conditions led to the formation of several types of nanostructures [40] . In the present study, mixtures of nanosheets, nanostripes, nanofibres, nanodroplets and nanoparticles were spontaneously observed in different proportions from dissociated spider silk fibres in water (see Supplementary Fig. 8 ). The size and shape of such nanocomposites were strongly species-dependent and related to the presence and proportion of the different subgroups of spidroins or even their intrinsic structural features (see Supplementary Fig. 9 ). To avoid any risk of analysing fibres that were not dragline silks or their equivalent, the molecular identity of the spidroins from species with available cDNA sequences ( Ajur , Ncla , Ncru and Pbis ) was confirmed by de novo sequencing of proteolytic peptides generated from dissociated silks (see Supplementary Fig. 10 ). Spider silk fibres resistance over temperature and proteases Consistent with the singular mechanostructural features of the natural silk fibres, the dissociated spidroins were thermally stable to at least 100 °C (see Supplementary Fig. 11a–c ) and were time-dependently resistant to proteolytic cleavage, with the exception of enzymes with promiscuous hydrolytic specificity that were used to confirm identities (see Supplementary Figs 11d–l and 12 ). Despite a growing body of evidence on these singular features of spidroins, the precise molecular reason for such attributes compared with other proteins remains obscure. One potential mechanism is the cooperative hydrogen bonding pattern of the intra- and mainly inter-chains of the repetitive protein modules [3] , [41] . However, we are certain that other mechanisms are involved, including that responsible for stabilizing molecules encrusted in spider silk fibres, for example, lipids and other organic compounds (see Supplementary Fig. 13 ), or even metals. Validity of nanoscale phylogeny based on AFM data Humans are innate taxonomists, and this feature helps us better understand the inheritance relationships among organisms. Because taxonomic characteristics are any group of detectable attributes of an organism that can be used for diagnostics, we believe that AFM and molecular data not only enable the selection of motifs appropriate for synthetic biology but also permit the reconstruction of a spider’s life history. 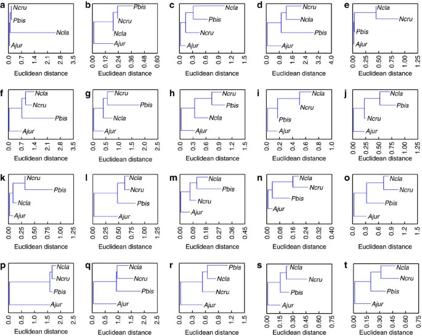Figure 5: Cladograms showing phylogenetic relationships. Cladograms demonstrating the phylogenetic relationships of spiders inferred using a diversity of theoretical or experimental characteristics. (a) Google engines search (Google web, Google scholar, Google images, Google videos, Google books, Google groups, Youtube), (b) diameter, (c) mass spectrometry, (d) cDNA codon usage, (e) elemental composition, (f) amino-acid composition, (g) physical-chemical, (h) protein motifs, (i) protein modules, (j) repeats, (k) palindromes, (l) secondary structure network protein sequence (NPS) consensus, (m) molecular modelling, (n) fourier transform infrared (FTIR) spectroscopy, (o) dissociated fibres, (p) nanoroughness-line profile, (q) nanoroughness-area, (r) nanoscale parameters, (s) nanomechanics-static, (t) nanomechanics-dynamic. Figure 5 summarizes our results for the four species for which structural and molecular data are available and shows that most of the present spider silk investigative approaches recapitulate the expected phylogeny of the species. Figure 5: Cladograms showing phylogenetic relationships. Cladograms demonstrating the phylogenetic relationships of spiders inferred using a diversity of theoretical or experimental characteristics. ( a ) Google engines search (Google web, Google scholar, Google images, Google videos, Google books, Google groups, Youtube), ( b ) diameter, ( c ) mass spectrometry, ( d ) cDNA codon usage, ( e ) elemental composition, ( f ) amino-acid composition, ( g ) physical-chemical, ( h ) protein motifs, ( i ) protein modules, ( j ) repeats, ( k ) palindromes, ( l ) secondary structure network protein sequence (NPS) consensus, ( m ) molecular modelling, ( n ) fourier transform infrared (FTIR) spectroscopy, ( o ) dissociated fibres, ( p ) nanoroughness-line profile, ( q ) nanoroughness-area, ( r ) nanoscale parameters, ( s ) nanomechanics-static, ( t ) nanomechanics-dynamic. Full size image To gain insight into the possible molecular reason for these facts, we previously sequenced cDNA products that represent spidroin coding regions from the silk glands of three evolutionarily unrelated spider species [42] and compared them with the best known spidroins from Nephila clavipes (see Supplementary Fig. 14 ). In this way, the semantic sequence comparison (see Supplementary Fig. 14a ), hierarchical amino-acid clustering (see Supplementary Fig. 14b ), relative amino-acid content (see Supplementary Fig. 14c ) and the specific-sequence repetitive domains (see Supplementary Fig. 14d ) signalled the molecular reasons for the mechanostructural facts observed in the present study. However, from a molecular viewpoint, a neglected feature of the spidroin protein sequences related to the recurrent presence of internal palindromes drew most of the attention even when compared with the presence of larger repeating units (see Supplementary Fig. 15 ). Palindromes are a ubiquitous feature of linguistics [43] , music [44] , mathematics [45] , computation [46] and biology [47] , [48] . The recurrence of palindromes in proteins represents a fundamental paradigm shift in structure-function studies because typical examples exhibit some kind of extraordinary feature [48] or undergo structural distortion under singular conditions [49] . Despite the uncertain contribution of the palindromes to the mechanostructural features observed in the present study, a systematic evaluation of their importance using synthetic biology approaches with recombinant spider silk proteins will be investigated further. The present experiments not only show that we and others can explore nanoscale patterns of spider silk fibres biodiversity using multiple modes of AFM experiments, but also that this conceptually novel approach can be used as a method to select, on demand, high-performance fibres that could be used as models for nanoengineering purposes. In view of the increasing demand for novel materials, this approach can be used when performing a reverse bioengineering process. In addition, this approach, with minor adaptations, can be applied to investigate nanoscale features of several other materials, including plastics, metals, ceramics, glasses, papers, woods and resins. Sample preparation Spider silks were supplied by Dr Paulo C. Motta (Institute of Biology, University of Brasilia, Brazil) and by Dr Randolph V. Lewis (Department of Molecular Biology, University of Wyoming, USA) and originated from spiders captured under IBAMA/MMA licence number (0128753 BR). Silks were reeled from adult specimens of Aglaoctenus lagotis (Araneomorphae, Lycosidae), Avicularia juruensis (Mygalomorphae, Theraphosidae), Avicularia species (Mygalomorphae, Theraphosidae), Argiope argentata (Araneomorphae, Araneidae), Argiope lobata (Araneomorphae, Araneidae), Gasteracantha cancriformis (Araneomorphae, Araneidae), Parawixia bistriata (Araneomorphae, Araneidae), N . clavipes (Araneomorphae, Nephilidae), Nephilengys cruentata (Araneomorphae, Tetragnathidae) and Pholcus phalangioides (Araneomorphae, Pholcidae). Silk fibres extruded from major ampullate gland spigots (or acinous gland spigots for Avicularia species) were rolled around a rotating tubular graphite at 5 mm s −1 , taking care to avoid contamination by silks that did not originate in the desired glands. Moreover, the assignments of the silk to the correct gland sources were confirmed by MALDI-TOF MS/MS analysis of proteolytically cleaved fragments of some AFM-analysed samples. Two synthetic fibres termed Recombinant-1 (MaSp-1, 16 × GGLGGQGGLGGLGSQGAGLGGYGQGGAGQGGAAAAAAAAS module, P. bistriata ) and Recombinant-2 (MaSp-2, 16 × GPGGYGPGQQGPGGYGPGQQGPSGPGSAAAAAAAA module, N . clavipes ) were expressed, purified and polymerized according to previously described methods [38] and deposited on a glass coverslip. Dissociated fibres were also deposited onto a freshly cleaved muscovite mica surface. Silk fibre samples were stored in a dust-free and light-protected petri dish under ambient conditions until analysis. Nylon and steel were used as controls. Multimode AFM analyses AFM was performed in contact, soft contact, force modulation, lateral force (trace-minus-retrace data), dynamic, phase imaging and KFM operation/acquisition modes on a SPM-9600 (Shimadzu, Japan) with suitable probes (see Supplementary Table 1 ) in a temperature-controlled room (23 °C) under atmospheric conditions. AFM scans of similar areas were acquired at a resolution of 512 × 512 pixels and a rate of 0.5–1 Hz. The scanned areas were perfect squares that ranged in size from 40 × 40 μm to 250 × 250 nm. We used four AFM off-line software packages to qualitatively and quantitatively analyse the acquired images (SPM-9600 off-line v. 3.304—Shimadzu, Japan; SPIP v. 5.1.5—Image Metrology, Denmark; WSxM v. 5.0 Develop 3.2—Nanotec Electronica, Spain; and Gwyddion v. 2.22—Czech Metrology Institute, Czech Republic). Quantitative nanoroughness, nanostiffness, nanofriction, nanoviscoelasticiy and nanopotential were acquired by measuring the RMS and the RSERMS of 15 images acquired at higher magnification of each sample for each mode, which totalled 1050 images. Unsupervised hierarchical clustering analysis was used to investigate the possibility of identifying subgroups in silk fibres based on their nanoscale features as measured by the RMS and RSERMS. Finally, this proposed multimode AFM method has also been proved feasible through the experimental data validation with literature data (see Supplementary Fig. 16 ). Single-fibre force spectroscopy analyses Force spectroscopy experiments were performed in ambient air with the same AFM-imaged fibres. The approach-release curves were recorded at 23 °C, 30% relative humidity, and a pulling rate of 1 Hz. Twelve force-distance curves were obtained from distinct regions from five different fibres. Data for the complete sample set were acquired with the same tip at the same AFM acquisition setup. Static and dynamic nanomechanics were determined using maximum load, maximum pull and snap in forces; detach separation and zero indentation distances; Young’s modulus; and energies dissipated. Ageing effect Fibres of five species were analysed by AFM operated under similar conditions after one year of storage to compare the results related to structural and mechanical features. Metal-binding effect Fibres of two phylogenetically distant species were investigated by force spectroscopy after incubation with Cu(II) and Pb(II) metal ions using the same measurement conditions and instrumental setup previously described. Mass spectrometric analyses Samples from the mechanically dissociated silk fibres digested in solution with aminopeptidase-M, carboxypeptidase-Y, chymotrypsin, elastase, endoproteinase Asp-N, endoproteinase Glu-C, endoproteinase Lys-C, proteinase-K and trypsin were desalted, concentrated and fractionated by in-tip reverse-phase chromatography (Zip-Tip C 18 , Millipore, USA) under increasing concentrations of acetonitrile (0, 10, 30, 50, 70, 90 and 100%). Mass spectra were obtained with an UltraFlex III MALDI-TOF/TOF mass spectrometer (Bruker Daltonics, Germany) operated in reflector, LIFT, CID and ISD modes under suitable conditions. De novo peptide sequences were obtained by manual interpretation of the MS/MS and ISD spectra. Sequence alignments and calculations Deduced protein sequences obtained from public and private cDNA libraries were searched for the recurrence of typical structural motifs, repeats and palindromes using an in-house Excel macro written in VBA. Sub-sequences that contained repeat motifs were submitted to multiple alignment comparisons using ClustalW running under BioEdit, and logos were drawn by WebLogo ( http://weblogo.berkeley.edu/logo.cgi ). Hydrophobic cluster analysis representations of the protein sequences were obtained from the DrawHCA server ( http://mobyle.rpbs.univ-paris-diderot.fr/cgi-bin/portal.py?form=HCA ) using the consensus sequences generated by WebLogo. The consensus secondary structures of conserved motifs were predicted using the Network Protein Sequence Analysis server ( http://pbil.ibcp.fr/ ). Automated homology modelling of the spidroins was performed on the ModWeb server ( http://modbase.compbio.ucsf.edu/ ). The conformers with the selected structures were subjected to energy minimization using the GROMOS 43B1 force field in the software Swiss-PdbViewer (version 4.1). The quality of the predicted structures was examined using WHATIF. All spidroin sequences data have been previously deposited in GenBank and are available under accession. Further methods and sequence codes can be obtained on request. Statistical analyses One-way ANOVA was used to compare data among groups followed by the Tukey’s multiple comparison post hoc test at a P <0.01 using PAST 2.17 software [50] . Multivariate data set comparisons were based on cluster (Euclidean distance) and principal component analyses of normalized data using PAST. How to cite this article: Silva, L. P. and Rech E. L. Unravelling the biodiversity of nanoscale signatures of spider silk fibres. Nat. Commun. 4:3014 doi: 10.1038/ncomms4014 (2013).